A role for TREX components in the release of spliced mRNA from nuclear speckle domains The TREX complex, which functions in mRNA export, is recruited to mRNA during splicing. Both the splicing machinery and the TREX complex are concentrated in 20–50 discrete foci known as nuclear speckle domains. In this study, we use a model system where DNA constructs are microinjected into HeLa cell nuclei, to follow the fates of the transcripts. We show that transcripts lacking functional splice sites, which are inefficiently exported, do not associate with nuclear speckle domains but are instead distributed throughout the nucleoplasm. In contrast, pre-mRNAs containing functional splice sites accumulate in nuclear speckles, and our data suggest that splicing occurs in these domains. When the TREX components UAP56 or Aly are knocked down, spliced mRNA, as well as total polyA+ RNA, accumulates in nuclear speckle domains. Together, our data raise the possibility that pre-mRNA undergoes splicing in nuclear speckle domains, before their release by TREX components for efficient export to the cytoplasm. Biochemical studies have revealed that the machineries for transcription, RNA processing and mRNA export are extensively coupled to one another via a complex network of both physical and functional interactions [1] , [2] , [3] , [4] . Coupling among the steps of gene expression is also apparent at the cellular level [4] , [5] , [6] . For example, in yeast, defects in either the factors or steps in mRNA processing typically result in accumulation of transcripts at the site of transcription where they are ultimately degraded [7] , [8] , [9] , [10] . Likewise, yeast transcripts are retained and degraded at the site of transcription in mRNA export mutants [10] . Although less is understood in human cells, several studies have raised the possibility that the coupled steps in gene expression take place within or near nuclear compartments variously known as nuclear speckle domains, splicing factor compartments, interchromatin granules or SC35 domains [4] , [5] . The earliest reports came from fluorescence in situ hybridisation (FISH) analysis of RNA transcripts from highly expressed endogenous genes [5] (and references therein). These studies indicated that, for many genes, transcription occurs in the vicinity of nuclear speckle domains and that mRNA processing occurs near or within the domains [11] , [12] , [13] , [14] , [15] . Additional work supported the view that nuclear speckle domains are sites of RNA processing, as evidence indicates that pre-mRNAs can undergo spliceosome assembly and splicing within nuclear speckle domains [5] , [16] , [17] , [18] , [19] , [20] . Recent studies have lent additional support to the view that nuclear speckle domains have an important role in the expression of actively transcribed genes [4] , [6] . In particular, an active allele or coexpressed genes cluster together around, or associate with, nuclear speckle domains [21] , [22] , [23] . For example, cotranscribed erythroid genes located on four different chromosomes cluster together around a common nuclear speckle domain [21] . Other studies of nuclear speckle domains indicate that they function as storage and recycling sites for the RNA processing machinery, and for some genes, the processing machinery moves from these domains to the transcriptionally active genes [24] , [25] , [26] , [27] , [28] . Additional work has also led to the view that nuclear speckle domains are sites where overexpressed exogenous pol II transcripts and/or aberrant RNAs (such as cDNA transcripts) accumulate [26] , [27] . However, other studies are not consistent with this view, as cDNA transcripts were not detected in nuclear speckle domains [18] , [19] , [20] . Thus, further work is needed to understand how nuclear speckle domains function in the pathway of gene expression. Nuclear speckle domains are not only the sites enriched in RNA processing machineries but also contain the mRNA export machinery (for example, the TREX complex) and mRNA surveillance machinery (for example, exon junction complex) [5] , [28] , [29] , [30] . The conserved TREX complex contains the multi-subunit THO complex and UAP56, Aly, Tex1 and CIP29 [31] , [32] , [33] , [34] , [35] , [36] (K.D., R.R., unpublished observation). In humans, efficient recruitment of the TREX complex to mRNA is splicing dependent, consistent with the observation that the TREX complex colocalizes with splicing factors in nuclear speckle domains [31] , [32] . Specifically, we previously found that the TREX complex is more efficiently recruited to mRNAs generated by splicing than to cDNA transcripts [37] , [38] , [39] , [40] . This increased recruitment correlated with increased export efficiency of spliced mRNAs relative to cDNA transcripts [41] . During this analysis [41] , we observed that the transcripts containing introns were present in discrete nuclear foci in HeLa cells, but this observation was not further investigated. In this study, we have used a nuclear microinjection assay to determine the fates of transcripts encoded by CMV-DNA constructs either containing or lacking functional splice sites. We show that both types of transcripts are detected at similar levels in the nucleus. However, cDNA transcripts and three different random-sequence transcripts do not associate with nuclear speckle domains, whereas transcripts containing functional splice sites do. Using splicing-specific FISH probes, our data suggest that splicing occurs in nuclear speckle domains. Finally, we show that a spliced reporter mRNA, as well as total polyA+ RNA, accumulates in nuclear speckle domains when TREX components UAP56 or Aly are knocked down. Together, these data indicate that transcripts containing functional splice sites associate with nuclear speckle domains, undergo splicing within these domains, and TREX components UAP56 and Aly function in releasing the mRNA from the domains for export to the cytoplasm. How these data relate to expression of endogenous genes is discussed. Splicing-dependent association of RNA with nuclear speckles We previously showed that spliced mRNAs are exported more efficiently than their corresponding cDNA transcript counterparts in both Xenopus oocytes and HeLa cells [41] , [42] . To further investigate the role of splicing in mRNA export, we microinjected a variety of DNA constructs containing a cytomegalovirus (CMV) promoter and the bovine growth hormone (BGH) polyadenylation site into HeLa cell nuclei and then examined the nucleocytoplasmic distribution of the transcripts using FISH. Initially, we compared a wild-type (WT) CMV-β-globin DNA construct containing its natural introns, a CMV-β-globin cDNA and three CMV-DNA constructs encoding random sequences lacking functional splice sites ( Fig. 1a ). Each of these constructs was microinjected into nuclei, cells were fixed after 5 min of incubation, followed by FISH ( Fig. 1b , inset panels show the dextran nuclear injection marker). This analysis revealed that all of the CMV constructs were transcribed and that the nascent transcripts were detected in the nucleus. Quantitation of FISH images for a minimum of 40 individual cells per construct revealed that the total amount of RNA detected was similar for all five constructs ( Fig. 1c ). Consistent with previous results [41] , by 6 hr after microinjection, spliced WT β-globin mRNA was largely detected in the cytoplasm, whereas the cDNA transcript and three random sequence transcripts were largely detected in the nucleus ( Supplementary Fig. S1 ). We conclude that both spliced and cDNA/random sequence RNAs are present at similar levels, and only the spliced mRNA accumulates at higher levels in the cytoplasm. 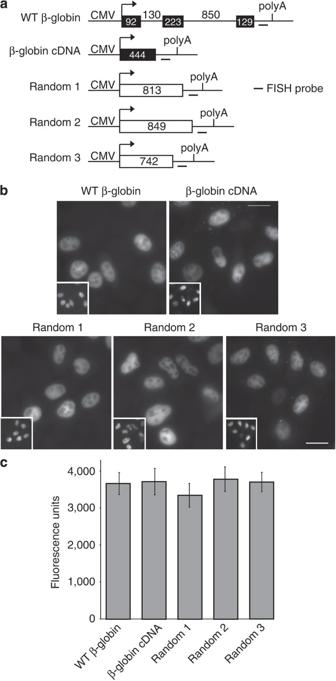Figure 1: FISH of RNAs after transcription of CMV-DNA constructs. (a) Schematic of constructs. The CMV promoter and BGH polyA sites and the location of the FISH probe (indicated by short line) are shown. The sizes (in nucleotides) of the introns, exons, cDNA and random transcripts are indicated for the respective constructs. (b) FISH of indicated transcripts that were detected 5 min after microinjection of CMV-DNA constructs (50 ng μl−1) into HeLa cell nuclei. FITC-conjugated dextran was coinjected as a nuclear marker (inset panels). Scale bar, 10 μm. (c) Quantification of total FISH fluorescence was determined for a minimum of 40 cells for each construct. Data represent the average of three experiments, and error bars indicate s.e. Figure 1: FISH of RNAs after transcription of CMV-DNA constructs. ( a ) Schematic of constructs. The CMV promoter and BGH polyA sites and the location of the FISH probe (indicated by short line) are shown. The sizes (in nucleotides) of the introns, exons, cDNA and random transcripts are indicated for the respective constructs. ( b ) FISH of indicated transcripts that were detected 5 min after microinjection of CMV-DNA constructs (50 ng μl −1 ) into HeLa cell nuclei. FITC-conjugated dextran was coinjected as a nuclear marker (inset panels). Scale bar, 10 μm. ( c ) Quantification of total FISH fluorescence was determined for a minimum of 40 cells for each construct. Data represent the average of three experiments, and error bars indicate s.e. Full size image To further investigate the distribution of WT β-globin transcripts, we microinjected the CMV-β-globin DNA construct, α-amanitin was added 30 min after microinjection, and then a time course was carried out using FISH. 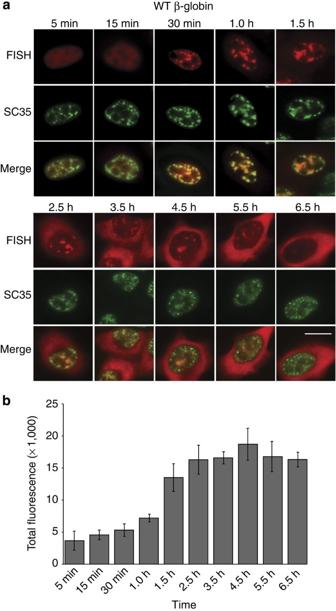Figure 2: WT β-globin transcripts associate with nuclear speckle domains. (a) FISH time course showing nucleocytoplasmic distribution of β-globin transcripts after microinjection of WT β-globin DNA construct into HeLa cell nuclei. α-amanitin was added at the 30-min time point to block further transcription. Cells were incubated for the indicated times before fixation. FISH, immunofluorescence (IF) using an SC35 monoclonal antibody and merged images are indicated. Scale bar, 10 μm. (b) Quantification of total FISH fluorescence was determined for a minimum of 10 cells for each time point. Data represent the average of three experiments, and error bars indicate s.e. A representative cell for each time point is shown in Figure 2a , and fields of cells are shown in Supplementary Figure S2 . As indicated by quantitation of the FISH signal ( Fig. 2b ), transcripts continued to accumulate for up to 1.5 h, most likely due to the time required for the α-amanatin to inhibit further transcription. Examination of the WT β-globin FISH signal at the 5- and 15-min time points revealed that the transcripts were evenly distributed throughout the nucleoplasm ( Fig. 2a , FISH panels). By 30 min, the transcripts began to concentrate as multiple nuclear foci and continued to be detected in these foci for up to 1.5 h ( Fig. 2a , FISH panels). Thereafter, the transcripts were also detected in the cytoplasm where they continued to accumulate over time ( Fig. 2a , FISH panels). As shown in Figure 2a (SC35 and merge panels), the nuclear foci containing the β-globin transcripts colocalize by immunofluorescence with the splicing factor SC35, the standard marker for nuclear speckle domains [4] , [5] , [28] . As our FISH assay detects RNA transcripts as a population, and previous work has shown that RNA and the contents of nuclear speckle domains move dynamically between the domains and the nucleoplasm [43] , our study does not distinguish between the (long debated) possibilities that nascent transcripts enter pre-existing nuclear speckle domains or whether factors exit the domains and associate with nascent transcripts to form speckles. A great deal of elegant work has dealt with these issues and also with the detailed morphology of nuclear speckle domains and sub-domains within nuclear speckle domains [5] , [44] (and references therein). In addition, previous work [17] and our study show that nuclear speckle domains often appear enlarged and/or coalesced, possibly because of the large amount of RNA associated with the domains under certain conditions. Our study is not focused on these detailed aspects of nuclear speckle domain formation, dynamics and morphology, and thus, with these caveats in mind, for simplicity, we will refer to transcripts as being in nuclear speckle domains throughout this manuscript. Figure 2: WT β-globin transcripts associate with nuclear speckle domains. ( a ) FISH time course showing nucleocytoplasmic distribution of β-globin transcripts after microinjection of WT β-globin DNA construct into HeLa cell nuclei. α-amanitin was added at the 30-min time point to block further transcription. Cells were incubated for the indicated times before fixation. FISH, immunofluorescence (IF) using an SC35 monoclonal antibody and merged images are indicated. Scale bar, 10 μm. ( b ) Quantification of total FISH fluorescence was determined for a minimum of 10 cells for each time point. Data represent the average of three experiments, and error bars indicate s.e. Full size image Importantly, quantitation of the total FISH signals during our time course ( Fig. 2b ) revealed that the β-globin transcripts remain at about the same levels starting at 1.5 h through 6.5 h. Over this time period, transcripts are detected in nuclear speckle domains and then detected in the cytoplasm. As the levels of transcripts were roughly the same over this time period, these data indicate that most of the RNA associated with the nuclear speckle domains is exported to the cytoplasm. Together, our data indicate that β-globin transcripts are at first present throughout the nucleoplasm at the earliest times after transcription, followed by association with nuclear speckle domains, and are then rapidly exported to the cytoplasm without an intermediate site of accumulation. Thus, transcript release from nuclear speckle domains appears to be a rate-limiting step in export of at least this spliced mRNA reporter. To further investigate the significance of the speckle association of WT β-globin transcripts ( Fig. 2 ), we microinjected three CMV-DNA constructs encoding random sequences and a construct encoding CMV-β-globin cDNA into HeLa cell nuclei, followed by addition of α-amanitin at 30 min ( Fig. 3a,b ). FISH analysis at the earliest time point after microinjection (5 min, Fig. 3a ) revealed that Random 1 transcripts were evenly distributed throughout the nucleoplasm, as observed with WT β-globin transcripts ( Fig. 2a ). However, in contrast to WT β-globin transcripts, Random 1 transcripts remained evenly distributed in the nucleoplasm throughout the time course ( Fig. 3a , FISH panels). Moreover, colocalisation studies with SC35 revealed that Random 1 transcripts do not associate with nuclear speckle domains ( Fig. 3a , SC35 and merge panels). A FISH comparison at the 1-h time point for all three Random transcripts and the β-globin cDNA transcript revealed that none of these transcripts colocalized with SC35 ( Fig. 3b ). Consistent with these data, a FISH time course carried out for Random 2 and 3 transcripts confirmed that they do not associate with nuclear speckle domains at any time point ( Supplementary Fig. S3 ). Finally, when another WT CMV-DNA construct, AdML, or a splice-defective counterpart containing mutated 5′ and 3′ splice sites (CMV-AdMLΔ5′Δ3′), was microinjected into HeLa cell nuclei, the WT AdML transcript was distributed in discrete nuclear foci, which colocalized with SC35 ( Fig. 3c , SC35 and merge) whereas the AdMLΔ5′Δ3′ transcript was diffusely distributed in the nucleoplasm ( Fig. 3c , SC35 and merge). Together, the data with all of our constructs indicate that association of transcripts with nuclear speckle domains requires functional splice sites. 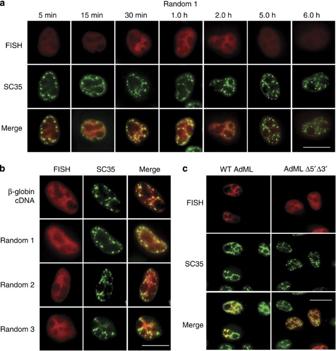Figure 3: Splice site-dependent association of transcripts with nuclear speckle domains. (a) CMV Random 1 DNA construct was microinjected into HeLa nuclei, and α-amanitin was added after 30 min to block further transcription. A FISH time course for Random 1 RNA was carried out at the indicated times. FISH, IF using an SC35 monoclonal antibody and merged images are shown. Scale bar, 10 μm. (b) Same asaexcept that Random 1, 2 and 3 CMV-DNA constructs and CMV β-globin cDNA construct were microinjected, and FISH was carried out 1 h after microinjection. (c) Same asaexcept that CMV-WT AdML or CMV-Δ5′Δ3′ AdML DNA constructs were used, and FISH was carried out 30 min after microinjection. FISH, IF using an SC35 monoclonal antibody and merged images are shown. Scale bar, 10 μm. Figure 3: Splice site-dependent association of transcripts with nuclear speckle domains. ( a ) CMV Random 1 DNA construct was microinjected into HeLa nuclei, and α-amanitin was added after 30 min to block further transcription. A FISH time course for Random 1 RNA was carried out at the indicated times. FISH, IF using an SC35 monoclonal antibody and merged images are shown. Scale bar, 10 μm. ( b ) Same as a except that Random 1, 2 and 3 CMV-DNA constructs and CMV β-globin cDNA construct were microinjected, and FISH was carried out 1 h after microinjection. ( c ) Same as a except that CMV-WT AdML or CMV-Δ5′Δ3′ AdML DNA constructs were used, and FISH was carried out 30 min after microinjection. FISH, IF using an SC35 monoclonal antibody and merged images are shown. Scale bar, 10 μm. Full size image We also investigated the nuclear localisation of the microinjected CMV-DNA constructs and found that they associated with nuclear speckle domains in a splice site-dependent manner ( Supplementary Fig. S4 ). The CMV-DNA constructs most likely move by free diffusion. The splice site-dependent association with nuclear speckle domains may occur because nascent transcripts with functional splice sites are still attached to the DNA. Further studies are needed to determine whether these observations with the CMV constructs are related to studies showing that actively transcribed endogenous genes associate with nuclear speckle domains [4] , [5] , [21] . Evidence that splicing occurs in nuclear speckle domains We next investigated whether splicing of the CMV transcripts occurs in nuclear speckle domains. Initially, we carried out reverse transcription (RT)–PCR to obtain a general idea about the splicing kinetics of the total β-globin RNA population after microinjection of the CMV-DNA construct. Mostly unspliced pre-mRNA was present at early times (5 and 15 min) after microinjection and mostly spliced mRNAs at later time points (30 and 60 min; Supplementary Fig. S5 ). We next carried out a FISH time course using a probe to the exon 2–exon 3 splice junction (SJ probe) to detect only spliced mRNA or a probe specific to intron 2 (intron probe, which detects both the unspliced pre-mRNA and the intron; Fig. 4 ). By 5 and 15 min after microinjection, β-globin RNA was detected throughout the nucleoplasm, and only with the intron probe ( Fig. 4 ), consistent with the presence of unspliced pre-mRNA at early times. By 30 min, the RNA was detected with both the SJ and intron probes, consistent with the presence of spliced mRNA at this time point. Of particular significance, the transcripts detected with the SJ and intron probes were well colocalized with each other, but were present in only a subset of nuclear speckle domains ( Fig. 4 , 30 min, compare SJ and intron probe panels and merge, and compare SJ/SC35 merge and intron/SC35 merge). The observation that the same subset of nuclear speckle domains was detected with both the intron and the SJ probes suggests that splicing occurs within the nuclear speckle domains. If, for example, the RNA was moving rapidly between different speckles, then we would expect to detect different speckles with the intron versus the SJ probe. 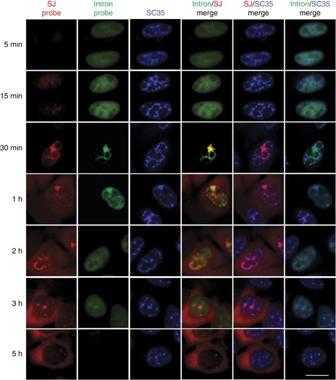Figure 4: FISH time course of β-globin transcripts using SJ- or intron-specific probes. CMV β-globin DNA construct was microinjected into nuclei, α-amanitin was added at 30 min and FISH was carried out at the indicated times. Probes were to the second SJ probe or the second intron (intron probe) of β-globin mRNA. IF was carried out using an SC35 monoclonal antibody. The indicated merged FISH and IF images are shown. Scale bar, 10 μm. Figure 4: FISH time course of β-globin transcripts using SJ- or intron-specific probes. CMV β-globin DNA construct was microinjected into nuclei, α-amanitin was added at 30 min and FISH was carried out at the indicated times. Probes were to the second SJ probe or the second intron (intron probe) of β-globin mRNA. IF was carried out using an SC35 monoclonal antibody. The indicated merged FISH and IF images are shown. Scale bar, 10 μm. Full size image To further investigate the possibility that splicing takes place within nuclear speckle domains, we carried out confocal microscopic analysis using the SJ probe as well as a probe to the exon–intron junction (EI probe, which detects unspliced pre-mRNA; Fig. 5a ). At the 30-min time point, the confocal data show that the transcripts detected with both the SJ and EI probes colocalize with each other and also with SC35. Moreover, the data show that the transcripts are localized in only a subset of the nuclear speckle domains. Z-stack confocal images further show the colocalisation of transcripts detected with the SJ and EI probes ( Fig. 5b ). Together, these data suggest that splicing of β-globin pre-mRNA occurs within nuclear speckle domains. 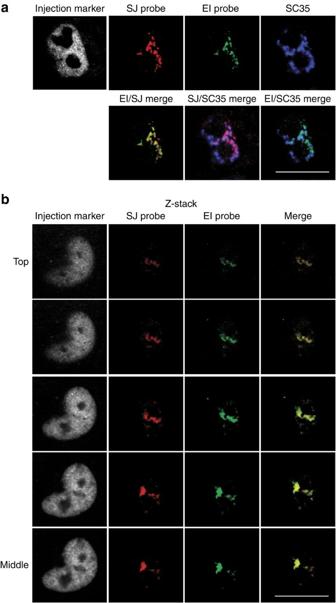Figure 5: Evidence that β-globin pre-mRNA is spliced in a subset of nuclear speckle domains. (a) CMV β-globin DNA was microinjected into nuclei, and FISH was carried out after 30 min using a probe to the SJ probe or the EI probe. IF with SC35 monoclonal antibody was carried out after the FISH. Confocal microscopy was used to visualize the cells. The nucleus was detected by the injection marker. The indicated merged images are shown in the second row. Scale bar, 10 μm. (b) Z-stacked confocal images for a representative nucleus using the indicated probes or SC35 antibody for IF are indicated. Z-stacks were taken in steps of micrometer. The top to middle sections of the Z-stacks are shown. Scale bar, 10 μm. Figure 5: Evidence that β-globin pre-mRNA is spliced in a subset of nuclear speckle domains. ( a ) CMV β-globin DNA was microinjected into nuclei, and FISH was carried out after 30 min using a probe to the SJ probe or the EI probe. IF with SC35 monoclonal antibody was carried out after the FISH. Confocal microscopy was used to visualize the cells. The nucleus was detected by the injection marker. The indicated merged images are shown in the second row. Scale bar, 10 μm. ( b ) Z-stacked confocal images for a representative nucleus using the indicated probes or SC35 antibody for IF are indicated. Z-stacks were taken in steps of micrometer. The top to middle sections of the Z-stacks are shown. Scale bar, 10 μm. Full size image UAP56 functions in release of mRNA from nuclear speckles As the TREX export machinery localizes in nuclear speckle domains and associates with mRNAs during splicing, we next investigated the link between TREX, mRNA export and nuclear speckle domains. Previous studies showed that UAP56 knockdown results in strong nuclear retention of mRNA with accumulation in distinct nuclear foci [45] , [46] , but the identity of these foci was not investigated. To characterize the foci, we carried out RNA-mediated interference (RNAi) of UAP56 in HeLa cells, using non-targeting short interfering RNAs (siRNAs) as a negative control. As shown by western blot analysis, UAP56 protein levels were efficiently knocked down ( Fig. 6a ). To determine the effects of the knockdown on the nucleocytoplasmic distribution of RNA, we microinjected the WT CMV-β-globin DNA construct ( Fig. 1a ) into HeLa cell nuclei, allowed transcription for 30 min, added α-amanitin to block further transcription and then used FISH to detect β-globin RNA after 3.5 h ( Fig. 6b ). In the negative control knockdown, β-globin RNA was detected mainly in the cytoplasm ( Fig. 6b , control (cntl) RNAi). In marked contrast, in the UAP56 knock down, β-globin RNA was detected in discrete nuclear foci ( Fig. 6b , UAP56 RNAi; a field of microinjected cells at lower magnification is shown in Fig. 6c ). 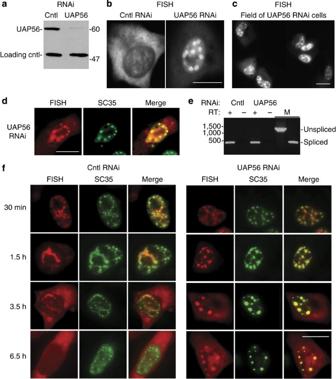Figure 6: β-Globin mRNA accumulates in nuclear speckle domains in UAP56 knockdown cells. (a) Western blot analysis using whole-cell lysates from cntl or UAP56 knockdown cells probed with an antibody against UAP56 or an antibody against tubulin as a loading control. Molecular weight markers in kilodaltons are shown. (b) CMV β-globin DNA construct was microinjected into the nuclei of control knockdown or UAP56 knockdown cells followed by FISH for β-globin mRNA. Scale bar, 10 μm. (c) Same asb, but shown at lower magnification. Scale bar, 10 μm. (d) FISH for β-globin mRNA in UAP56 knockdown cells 3.5 h after microinjection, SC35 IF using an SC35 monoclonal antibody, and merged FISH and IF images are shown. Scale bar, 10 μm. (e) RT–PCR of total RNA extracted from control knockdown and UAP56 knockdown cells microinjected with β-globin DNA. RT: + and − indicates reactions carried out in the presence or absence of RT, followed by PCR. DNA size markers (in base pairs) are indicated on the left. M: marker for unspliced and spliced mRNAs. (f) FISH time course showing nucleocytoplasmic distribution of β-globin transcripts after microinjection of WT β-globin DNA construct into the nuclei of control knockdown or UAP56 knockdown cells. α-Amanitin was added at the 30-min time point to block further transcription. Cells were incubated for the indicated times before fixation. FISH, IF using an SC35 monoclonal antibody, and merged FISH and IF images are shown. Scale bar, 10 μm. As shown in Figure 6d , the β-globin RNA detected by FISH colocalized with SC35. Thus, UAP56 knock down results in a strong accumulation of β-globin RNA in nuclear speckle domains. As immunodepletion of UAP56 in nuclear extracts results in inhibition of splicing in vitro [47] , [48] , and as splicing-defective transcripts that are capable of at least partial spliceosome assembly accumulate in nuclear speckle domains [5] , [16] (and references therein), we asked whether UAP56 knock down affected splicing of the β-globin reporter in vivo . As shown in Figure 6e , RT–PCR revealed only spliced mRNA in both the UAP56 knockdown and negative control knockdown cells. These data indicate that a splicing defect does not account for the accumulation of β-globin mRNA in nuclear speckle domains in the UAP56 knockdown cells. Figure 6: β-Globin mRNA accumulates in nuclear speckle domains in UAP56 knockdown cells. ( a ) Western blot analysis using whole-cell lysates from cntl or UAP56 knockdown cells probed with an antibody against UAP56 or an antibody against tubulin as a loading control. Molecular weight markers in kilodaltons are shown. ( b ) CMV β-globin DNA construct was microinjected into the nuclei of control knockdown or UAP56 knockdown cells followed by FISH for β-globin mRNA. Scale bar, 10 μm. ( c ) Same as b , but shown at lower magnification. Scale bar, 10 μm. ( d ) FISH for β-globin mRNA in UAP56 knockdown cells 3.5 h after microinjection, SC35 IF using an SC35 monoclonal antibody, and merged FISH and IF images are shown. Scale bar, 10 μm. ( e ) RT–PCR of total RNA extracted from control knockdown and UAP56 knockdown cells microinjected with β-globin DNA. RT: + and − indicates reactions carried out in the presence or absence of RT, followed by PCR. DNA size markers (in base pairs) are indicated on the left. M: marker for unspliced and spliced mRNAs. ( f ) FISH time course showing nucleocytoplasmic distribution of β-globin transcripts after microinjection of WT β-globin DNA construct into the nuclei of control knockdown or UAP56 knockdown cells. α-Amanitin was added at the 30-min time point to block further transcription. Cells were incubated for the indicated times before fixation. FISH, IF using an SC35 monoclonal antibody, and merged FISH and IF images are shown. Scale bar, 10 μm. Full size image To further examine the role of UAP56 in the accumulation of mRNA in nuclear speckle domains, we microinjected the CMV-β-globin DNA construct into UAP56 or control knockdown cells and then carried out a time course. At 30 min after microinjection, the accumulation of β-globin transcripts in nuclear speckle domains appeared similar in UAP56 and control knockdown cells ( Fig. 6f , 30 min). However, at subsequent time points, the nuclear speckle domains appeared rounded in the UAP56 knockdown cells compared with the control cells ( Fig. 6f ). This round phenotype likely results from the high levels of transcripts that accumulate in nuclear speckle domains in the UAP56 knockdown cells; these transcripts are able to exit the domains in the control knockdown (or normal) cells. The time course also shows that some of the β-globin mRNA reaches the cytoplasm by 3.5 and 6.5 h time points in the UAP56 knockdown cells ( Fig. 6f ). This may occur because sufficient UAP56 remains after knock down to allow the slow release from nuclear speckle domains (that is, a leaky phenotype) or because UAP56 knockdown only delays the release of mRNA from the domains. At present, we cannot distinguish between these and other possibilities. To ascertain whether UAP56-dependent release of spliced mRNAs from nuclear speckle domains occurs with endogenous mRNAs, we next examined the distribution of total polyA+ RNA in UAP56 knockdown cells. The expected distribution of polyA+ RNA was observed in negative control knockdown cells ( Fig. 7a , cntl RNAi), in which the RNA is present in both the nucleus and the cytoplasm [49] , [50] , [51] . In the nucleus, a portion of the steady-state polyA+ RNA is present in nuclear speckle domains [15] , [16] , [52] , [53] . In marked contrast to the non-knockdown cells, in the UAP56 knockdown cells, polyA+ RNA was only present in the nucleus where it strongly accumulated in multiple foci ( Fig. 7a , UAP56 RNAi). 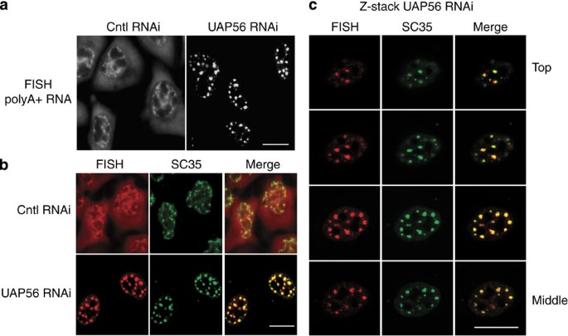Figure 7: PolyA+ RNA accumulates in nuclear speckle domains in UAP56 knockdown cells. (a) FISH of polyA+ RNA in control and UAP56 knockdown cells. Scale bar, 10 μm. (b) FISH for polyA+ RNA followed by IF using an SC35 monoclonal antibody in control or UAP56 knockdown cells. The merged FISH and IF images are shown in the right panel. Scale bar, 10 μm. (c) Z-stack confocal analysis of FISH for polyA+ RNA, SC35 IF and merged images are indicated. Z-stacks were taken in steps of micrometer. The top to middle sections of the Z-stacks are shown. Scale bar, 10 μm. As shown in Figure 7b , the polyA+ RNA in UAP56 knockdown cells colocalized with SC35, indicating that these foci correspond to nuclear speckle domains. Z-stack images from confocal microscopy confirm the colocalisation of polyA+ RNA in UAP56 knockdown cells with nuclear speckle domains ( Fig. 7c ). We conclude that UAP56 knock down results in the accumulation of polyA+ RNA in nuclear speckle domains. We did not detect any splicing defects in UAP56 knockdown cells when we assayed two endogenous mRNAs (DNAJB1 and BRD2, data not shown) [54] . Thus, as observed with β-globin mRNA, our data indicate that splicing inhibition is not likely to account for the accumulation of polyA+ RNA in nuclear speckle domains in UAP56 knockdown cells, though we cannot rule out the possibility that UAP56 knockdown inhibits splicing of a subset of pre-mRNAs. Figure 7: PolyA+ RNA accumulates in nuclear speckle domains in UAP56 knockdown cells. ( a ) FISH of polyA+ RNA in control and UAP56 knockdown cells. Scale bar, 10 μm. ( b ) FISH for polyA+ RNA followed by IF using an SC35 monoclonal antibody in control or UAP56 knockdown cells. The merged FISH and IF images are shown in the right panel. Scale bar, 10 μm. ( c ) Z-stack confocal analysis of FISH for polyA+ RNA, SC35 IF and merged images are indicated. Z-stacks were taken in steps of micrometer. The top to middle sections of the Z-stacks are shown. Scale bar, 10 μm. Full size image Aly functions in the release of mRNA from nuclear speckles To determine whether other TREX components have a role in the release of mRNA from nuclear speckle domains, we knocked down Aly ( Fig. 8a ). Consistent with previous studies [55] , [56] , Aly knock down inhibits mRNA export ( Fig. 8b ). Significantly, our data show that total polyA+ RNA is retained in nuclear speckle domains after Aly knock down ( Fig. 8b ). Z-stack images from confocal microscopy confirm the colocalisation of polyA+ RNA in Aly knockdown cells with nuclear speckle domains ( Fig. 8c ). Together, these data indicate that at least two TREX components, UAP56 and Aly, function in release of mRNA from nuclear speckle domains. 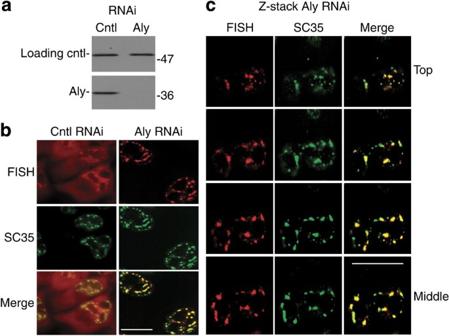Figure 8: PolyA+ RNA accumulates in nuclear speckle domains in Aly knockdown cells. (a) Western analysis using whole-cell lysates from cntl or Aly knockdown cells probed with an antibody against Aly or against tubulin as a loading control. Molecular weight markers in kilodaltons are shown. (b) FISH for polyA+ RNA followed by IF using an SC35 monoclonal antibody in control or Aly knockdown cells. The merged FISH and IF images are shown in the bottom panels. Scale bar, 10 μm. (c) Z-stack confocal analysis of FISH for polyA+ RNA, SC35 IF and merged images are indicated. Z-stacks were taken in steps of micrometer. The top to middle sections of the Z-stacks are shown. Scale bar, 10 μm. Figure 8: PolyA+ RNA accumulates in nuclear speckle domains in Aly knockdown cells. ( a ) Western analysis using whole-cell lysates from cntl or Aly knockdown cells probed with an antibody against Aly or against tubulin as a loading control. Molecular weight markers in kilodaltons are shown. ( b ) FISH for polyA+ RNA followed by IF using an SC35 monoclonal antibody in control or Aly knockdown cells. The merged FISH and IF images are shown in the bottom panels. Scale bar, 10 μm. ( c ) Z-stack confocal analysis of FISH for polyA+ RNA, SC35 IF and merged images are indicated. Z-stacks were taken in steps of micrometer. The top to middle sections of the Z-stacks are shown. Scale bar, 10 μm. Full size image Nuclear speckle domains are 25–50 discrete foci that contain the machineries for pre-mRNA processing and mRNA export (the TREX complex), as well as polyA+ RNA. In this study, we analyzed total polyA+ RNA and also microinjected CMV-DNA constructs into HeLa cell nuclei to investigate the relationships between pre-mRNA splicing, mRNA export and nuclear speckle domains. Our study led to three main conclusions. (1) Only pre-mRNAs containing functional splice sites localize to nuclear speckle domains. (2) Spliced mRNA accumulates within the domains. (3) The TREX components, UAP56 and Aly, function in releasing spliced mRNA/polyA+ RNA from the domains for export to the cytoplasm. As our work employed CMV-DNA constructs, which are introduced exogenously into nuclei and are also highly expressed, a key issue is how these data relate to expression of endogenous genes. An important point in this regard is that knockdown of TREX components resulted in the accumulation of not only the exogenous reporter mRNA, but also endogenous polyA+ RNA, in nuclear speckle domains. In contrast, we did not observe an increase in levels of polyA+ RNA in the surrounding nucleoplasm. Thus, these data raise the possibility that a significant fraction of the endogenous mRNA in the nucleus passes through nuclear speckle domains before export to the cytoplasm. As our data and previous work [18] , [19] indicate that association of transcripts with nuclear speckle domains is splicing dependent, the data argue that this fraction of endogenous mRNAs was spliced in nuclear speckle domains and then exported. Our study also shows that transcripts such as cDNAs or random-sequence RNAs do not associate with speckles, and these RNAs are poorly exported. Thus, putting all of the data together, it is possible that a pre-requisite for efficient export of many mRNAs is that pre-mRNAs enter nuclear speckle domains, undergo splicing, followed by TREX-dependent release and efficient export. Previous work has shown that splicing-defective introns that are either capable of forming partial spliceosomes or are part of multi-intron pre-mRNAs are retained in nuclear speckle domains [16] . Thus, these data indicate that nuclear speckle domains may function as quality control centres once these defective mRNAs are present in the domains [5] , [16] . Properly processed mRNAs that pass this quality control checkpoint are rapidly and efficiently exported. Recent studies showing that an active allele [23] , a set of hormone-regulated genes [22] or a set of regulated erythroid genes [21] all associate with nuclear speckle domains supports the view that these domains are specific sites for orchestrating nuclear events in the expression of at least a subset of genes [5] , [16] . In light of these studies on specific endogenous genes and our results, it will be interesting to determine the generality of nuclear speckle domain function in splicing and TREX-dependent release for export of endogenous pre-mRNAs. This analysis is especially relevant to previous studies indicating that splicing of at least some endogenous pre-mRNAs occurs at the site of transcription, and not within speckles [16] , [57] . Further work is needed to determine how these pre-mRNAs are targeted for export and why they do not increase in levels in the nucleoplasm when TREX components are knocked down. Although our data indicate that a key function for UAP56 and Aly, and possibly the entire TREX complex, is releasing spliced mRNA from nuclear speckle domains, further studies are needed to understand the mechanisms involved in this release as well as other important roles the TREX machinery may have during the mRNA export pathway. Molecular biology and antibodies The plasmids encoding WT human β-globin pre-mRNA and cDNA were constructed by adding a 5′ Myc tag and a 3′ HA tag to both intron-containing and intron-lacking β-globin by PCR amplification using the forward primer 5′-CGGGGTACCGCCGCCACCATGGAACAAAAACTCATCTCAGAAGAGGATCTGCCATGGGTGCATCTGACTCCT-3′ and the reverse primer 5′-CGCAGAGATATCTTAAGCGTAGTCTGGGACGTCGTATGGGTACGTAGCGTGATACTTGTGGGC-3′. PCR products were cloned into Kpn I and Eco RV sites in pcDNA3. The plasmids encoding CMV WT AdML and CMV Δ5′Δ3′AdML were constructed by inserting a PCR fragment containing AdML [58] and Δ5′Δ3′AdML [58] into the Kpn 1 and Xba 1 sites in pcDNA3.1. In the Δ5′Δ3′AdML [58] , the WT 5′ splice site sequence (GTTGGGGTGAG) was replaced with (ATTGGAGCCAC), and for the 3′ splice site mutation, eight consecutive T residues (nucleotides 155–162 in AdML) were replaced with GTGATCAC. The plasmid encoding Random 1 was constructed by using PCR to amplify a fragment from total genomic HeLa DNA containing the anti-sense sequence of human α-interferon ( IFNA1 ). The forward primer was 5′-ACTAAGCTTAGAACCTAGAGCCCAAGGTT-3′ and the reverse primer was 5′-ACTAAGCTTACACTAACCACAGTGTAAAGGT-3′. The PCR product was inserted into the Hin dIII site of pcDNA3. The plasmid encoding Random 2 was constructed by first inserting a PCR fragment containing the sense sequence of human βinterferon ( IFNB1 ) generated using the forward primer 5′-ACTGCTAGCACATTCTAACTGCAACCTTTCG-3′ and the reverse primer 5′-ACTCTTAAGCACAGCAGTTCATGCCAT-3′ into the Nhe 1/ Af1 II sites of pEGFP-N2. A PCR fragment containing the anti-sense sequence of this construct was then generated using the forward primer 5′-ACTGCTAGCAATACGACTCACTATAGGCAAGCTTACATTCTAACTGCAACCT-3′ and the reverse primer 5′-ACTAAGCTTTTCCAAAATAAAATTTAAAT-3′. This PCR product was subsequently inserted into the Hin dIII site of pcDNA3. The plasmid encoding Random 3 was constructed by first amplifying the sense sequence of human heat-shock protein B3 ( HSPB3 ) gene with the forward primer 5′-ATGCCCTATAAATAGCCGTTCATT-3′ and the reverse primer 5′-GCTGGCATTGTTGGAATAATAAGA-3′. Subsequently, a PCR fragment containing the anti-sense sequence of this construct was generated using the forward primer 5′-ATAGGGCCCGCATTCCGTGCTATGATTCA-3′ and the reverse primer 5′-GACGGTACCCTTCATAAAAATCATAGCAAAT-3′. This PCR product was inserted into the Kpn I and Apa I sites of pcDNA3. RT–PCR was used to detect spliced and unspliced β-globin RNA. The forward and reverse primers used for RT–PCR were 5′-ATGGTGCACCTGACTCCTGA-3′ and 5′-CACCAGCCACCACTTTCTGA-3′, respectively. To generate markers for unspliced and spliced β-globin RNA, these forward and reverse primers were used for PCR of WT or cDNA β-globin DNA constructs. For western blots, the UAP56 rabbit polyclonal antibody, which cross-reacts with its >90% identical relative URH49 [45] , [46] , was raised against full-length GST-UAP56 [40] and used at a dilution of 1:1,000. The Aly rabbit polyclonal antibody was raised against full-length GST-Aly and used at a dilution of 1:1,000. The tubulin monoclonal antibody was obtained from Sigma and used at a dilution of 1:1,000. Cell culture and RNAi HeLa cells were transfected with siRNAs using lipofectamine 2000 (Invitrogen) on 35-mm dishes with glass coverslip bottoms (MatTek Corp.). The siRNA target sequences for URH49 and UAP56 were 5′-AAAGGCCUAGCCAUCACUUUU-3′ and 5′-AAGGGCUUGGCUAUCACAUUU-3′, respectively [46] (it is of note that both UAP56 and its >90% identical homologue URH49 must be knocked down to observe a robust export block [45] , [46] ). The control non-targeting siRNA was purchased from Dharmacon (catalogue # D-001810-04-20). DNA microinjections and detection HeLa cells used for microinjection were plated on fibronectin-coated 35-mm dishes with glass coverslip bottoms (MatTek) [41] . Plasmid DNA (50 ng μl −1 ) was coinjected with FITC-conjugated 70-kDa dextran (Molecular Probes) [41] . In each experiment, 50–70 cells were microinjected, followed by incubation at 37 °C [41] . After 30 min of incubation, α-amanitin (50 μg ml −1 ) was added, and incubation was continued for the indicated times. A 70 bp FISH probe 5′-AAGGCACGGGGGAGGGGCAAACAACAGATGGCTGGCAACTAGAAGGCACAGTCGAGGCTGATCAGCGGGT-3′ that hybridizes to pcDNA 3.1 vector sequence was labelled at the 5′ end with Alexa Fluor 546 NHS Ester and high-performance liquid chromatography purified. For β-globin splicing assays, probes corresponding to splicing junction 2 (SJ probe) 5′-CACAGACCAGCACGTTGCCCAGGAGCCTGAAGTTCTCAGGATCCACGTGC-3′, exon 3–intron 2 junction (EI probe) 5′-CACAGACCAGCACGTTGCCCAGGAGCTGTGGGAGGAAGATAAGAGGTATG-3′, and intron 2 (intron probe) 5′-ATTCCAAATAGTAATGTACTAGGCAGACTGTGTAAAGTTTTTTTTTAAGTTACTTAATGT-3′ were labelled with ULYSIS Alexa Fluor nucleic acid labelling kits 647, 546 and 546, respectively (Invitrogen). For FISH to detect RNAs generated from microinjected CMV-DNA constructs, HeLa cells were fixed with 4% paraformaldehyde in PBS for 15 min and permeabilized with 0.1% Triton X-100 in PBS for 15 min [41] . Cells were then washed with 50% formamide in 1× SSC and incubated at 37 °C with FISH probes for 24 h [41] . For FISH to detect polyA+ RNA, an high-performance liquid chromatography-purified oligo dT(70) probe labelled at the 5′ end with Alexa Fluor 546 NHS Ester was used. HeLa cells were washed once with PBS, fixed for 10 min with 4% paraformaldehyde, washed three times with PBS, permeabilized with 0.5% Triton X-100 for 5 min, washed twice with PBS and then once with 2× SSC for 10 min at room temperature. The oligo dT(70) probe was then added at 1 ng μl −1 followed by incubation for 16–24 h at 42 °C. The cells were washed for 15 min each, twice with 2× SSC, once with 0.5× SSC and once with PBS at room temperature. Images were captured with an EM-CCD camera on an inverted microscope (200M; Zeiss) or a Nikon Ti w/Spinning Disk Confocal microscope using Metamorph software (Molecular Devices). FISH quantitation was carried out using imageJ 1.33u software (National Institutes of Health) [41] . For detecting CMV-DNA constructs after microinjection into HeLa cells, PCR constructs were generated using 5′Alexa-647 labelled forward primer 5′-TGGAGGTCGCTGAGTAGTGC-3′ and reverse primer 5′-CCACACCCTAACTGACAC-3′. Alexa-647 labelled PCR products were microinjected at a concentration of 50 ng μl −1 . Immunofluorescence was performed by incubating fixed cells with primary antibody for 30 min at room temperature. After washing three times in PBS for 10 min each, cells were incubated with the secondary antibody for 30 min at room temperature, followed by three washes in PBS for 10 min each. The SC35 primary antibody (Sigma) was diluted to 1:1,000 using 10% calf serum in PBS. The Mouse Alexa-647 (1:1,000), mouse Alexa-555 (1:1,000) and mouse Alexa-350 (1:50; Invitrogen) secondary antibodies were diluted into 10% calf serum. How to cite this article: Dias, A. P. et al . A role for TREX components in the release of spliced mRNA from nuclear speckle domains. Nat. Commun. 1:97 doi: 10.1038/ncomms1103 (2010).